Two new susceptibility loci 1q24.2 and 11p11.2 confer risk to severe acne Severe acne is a chronic inflammatory skin disorder characterized by widespread inflammatory lesions including nodules, cysts and potential scarring. Here we perform the first genome-wide association study of severe acne in a Chinese Han population comprising 1,056 cases and 1,056 controls using the Illumina HumanOmniZhongHua-8 BeadChip. In an independent cohort of 1,860 cases and 3,660 controls of Chinese Han, we replicate 101 SNPs of which 3 showed consistent association. We identify two new susceptibility loci at 11p11.2 ( DDB2 , rs747650, P combined =4.41 × 10 −9 and rs1060573, P combined =1.28 × 10 −8 ) and 1q24.2 ( SELL , rs7531806, P combined =1.20 × 10 −8 ) that are involved in androgen metabolism, inflammation processes and scar formation in severe acne. These results point to new genetic susceptibility factors and suggest several new biological pathways related to severe acne. Acne vulgaris is a common skin disease characterized by chronic inflammation of the pilosebaceous unit resulting from androgen-induced increased sebum production, altered keratinisation, inflammation and bacterial colonization of hair follicles by Propionibacterium acnes [1] . The prevalence of acne varies by age and ethnicity [2] , [3] , [4] . A community-based study performed in China found that acne was present in subjects older than 10 years of age and that the prevalence increased rapidly with age up to 46.8% in the19-year-old group [5] . In subjects with acne, 68.4% had mild (grade I acne of Pillsbury Grade [6] ), 26.0% had moderate (grade II and III) and 5.6% had severe acne (grade IV) [5] . Severe acne is characterized by widespread inflammatory lesions, such as nodules, cysts and potential scarring, often creating social handicaps and psychological problems [7] . Increasing evidence from large families and twins implicates genetic factors in the pathogenesis of acne [8] , [9] . Several candidate genes have thus far been implicated, which include tumour necrosis factor ( TNF) [10] , [11] , tumour necrosis factor receptor 2 ( TNFR2) [12] , toll-like receptor 2 ( TLR2) [12] , interleukin 1-alpha ( IL-1 α) [13] , cytochrome P450 family 1 subfamily A polypeptide 1 ( CYP1A1) [14] , cytochrome P450 family 17 subfamily A polypeptide 1 ( CYP17A1) [15] , cytochrome P450 family 21 subfamily A polypeptide 2 (CYP21A2) [16] and androgen receptor ( AR) [17] . These genes affect two major cellular processes: regulation of steroid hormone metabolism and the innate immune functions of epidermal keratinocytes. However, candidate gene studies were only carried out on small size cohorts, and no previous GWAS of acne has been published. The underlying genetic basis of acne remains poorly understood. Here we carry out a two-stage GWAS of severe acne involving 2,916 cases and 4,716 controls from a Chinese population to identify susceptibility loci/genes for severe acne. We identify two susceptibility loci at 11p11.2 and 1q24.2 that implicate genes related to androgen metabolism, inflammation processes and scar formation, suggesting their potential involvement in the aetiology of severe acne. 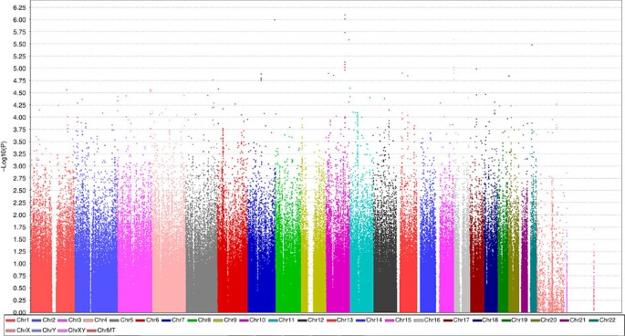Figure 1: Genome-wide association results from the GWAS analysis. The genome-wideP-values of the logistic regression test from 809,305 polymorphic SNPs in 1,031 severe acne cases and 1,031 control subjects of Chinese Han descent are presented. The chromosomal distribution of all theP-values (−log10P) is shown. GWAS association results In the discovery stage, we genotyped 900,015 SNPs using Illumina HumanOmniZhongHua-8 BeadChip in 1,056 cases and 1,056 controls of Chinese Han ( Table 1 ). After quality control, 809,305 SNPs (average call rate>98% and MAF>1%) in 1,031 severe acne cases and 1,031 controls of Chinese Han were used in the GWAS discovery analysis. Table 1 Sample characteristics of cases with severe acne and controls. Full size table The scatter plot of P -values using logistic regression with adjustment for the gender is shown in Fig. 1 . Principal component analysis (PCA) indicated minimal overall inflation of the genome-wide statistical results ( λ GC =1.01) ( Fig. 2 , Supplementary Data 1 ). Moreover, the quantile–quantile plot displayed no global departure from the expected null distribution of P- values ( Fig. 3 ). Both of these results indicate negligible inflation of the genome-wide association signals caused by population stratification, further suggesting that the deviated tail of the P- values’ distribution reflects some true genetic associations with severe acne. We then carried out logistic regression analysis to assess the genotype–phenotype association. Figure 1: Genome-wide association results from the GWAS analysis. The genome-wide P- values of the logistic regression test from 809,305 polymorphic SNPs in 1,031 severe acne cases and 1,031 control subjects of Chinese Han descent are presented. The chromosomal distribution of all the P- values (−log 10 P ) is shown. 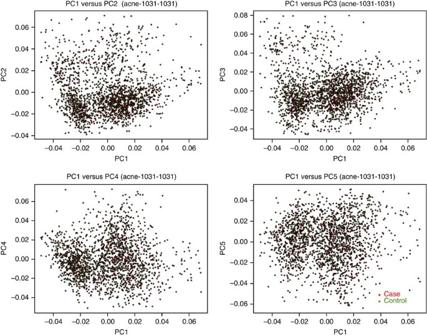Figure 2: Principal component analysis of GWAS samples. Principal component analyses (PCA) were performed in our 2,062 GWAS samples (1,031 cases and 1,031 controls). The case–control matching and the low lambda GC values (λGC=1.01) suggested minimal evidence of population stratification. Full size image Figure 2: Principal component analysis of GWAS samples. Principal component analyses (PCA) were performed in our 2,062 GWAS samples (1,031 cases and 1,031 controls). The case–control matching and the low lambda GC values ( λ GC =1.01) suggested minimal evidence of population stratification. 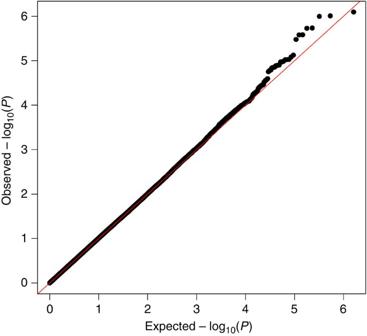Figure 3: Quantile–Quantile plots of the observedP-values for association in discovery stage. Purple points represent the distribution of logistic regressionP-values for the association of all the 809,305 SNPs in 1,031 cases and 1,031 control subjects of Chinese Han descent. Full size image Figure 3: Quantile–Quantile plots of the observed P -values for association in discovery stage. Purple points represent the distribution of logistic regression P- values for the association of all the 809,305 SNPs in 1,031 cases and 1,031 control subjects of Chinese Han descent. Full size image To perform a fast track replication study, we selected and genotyped 101 SNPs for replication in independent samples of 1,860 cases and 3,660 controls of Chinese Han ( Table 1 ). These SNPs included 86 SNPs with P <1 × 10 −4 in the discovery stage and 15 SNPs with nominal association evidence ( P <1 × 10 −2 in the discovery stage) located within or close to nine susceptibility genes that had gene expression profiling evidence for acne or three syndromes with acne symptoms (Apert syndrome, polycystic ovary syndrome and pyogenic arthritis, pyoderma gangrenosum and acne syndrome). After quality control, 87 SNPs remained for further replication analysis. In the replication stage, three of these SNPs showed consistent association in the independent replication samples and surpassed the threshold for Bonferroni correction in the validation analysis (rs747650, P =9.25 × 10 −6 , rs1060573, P =2.44 × 10 −5 , rs7531806, P =9.22 × 10 −7 ). All three SNPs at the two loci showed more significant association in the joint analysis of the combined discovery and replication samples: rs747650 and rs1060573 ( P combined =4.41 × 10 −9 , OR=1.24 and P combined =1.28 × 10 −8 , OR=1.23, respectively) at 11p11.2 ( DDB2) and rs7531806 ( P combined =1.20 × 10 −8 , OR=1.22) at 1q24.2 ( SELL ) ( Fig. 4 , Table 2 ). The SNPs identified in our GWAS did not situate in previously identified candidate genes, and no previously identified candidate genes were replicated in our study. The association results are shown in Supplementary Data 2 . 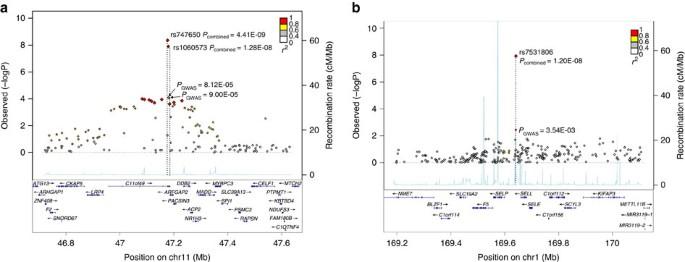Figure 4: Regional plots of two susceptibility loci for severe acne. (a) 11p11.2 and (b) 1q24.2. For each plot, the –log10P-values (lefty-axis) of SNPs are presented according to their chromosomal positions (x-axis). The top genotyped SNP is labeled by rs ID, and ther2-values of the rest of the SNPs with the top genotyped SNP are indicated by different colours. The genetic recombination rates (estimated using the HapMap Han Chinese in Beijing (CHB) and Japanese in Tokyo (JPT) samples) are represented by light blue lines. Genes within the region are annotated and shown as arrows.P-values were generated using logistic regression. Figure 4: Regional plots of two susceptibility loci for severe acne. ( a ) 11p11.2 and ( b ) 1q24.2. For each plot, the –log 10 P- values (left y- axis) of SNPs are presented according to their chromosomal positions ( x- axis). The top genotyped SNP is labeled by rs ID, and the r 2 -values of the rest of the SNPs with the top genotyped SNP are indicated by different colours. The genetic recombination rates (estimated using the HapMap Han Chinese in Beijing (CHB) and Japanese in Tokyo (JPT) samples) are represented by light blue lines. Genes within the region are annotated and shown as arrows. P -values were generated using logistic regression. Full size image Table 2 Significant association of three SNPs with severe acne risk. Full size table Analysis of different genetic models For the three significant SNPs, we used three different genetic models for further analysis: the dominant model, recessive model and additive model. Using a logistic regression analysis, we observed that the association of rs747650 and rs1060573 with severe acne under the additive model ( P =1.75 × 10 −9 and P =5.66 × 10 −9 , respectively) was more significant than under the dominant ( P =8.68 × 10 −9 and P =4.55 × 10 −8 , respectively) and recessive models ( P =2.07 × 10 −4 and P =1.89 × 10 −4 , respectively). Compared with A/A , the genotype of homozygote G/G (OR Hom =1.46 and OR Hom =1.45, respectively) showed larger OR than the heterozygote G/A (OR Het =1.28 and OR Het =1.25, respectively). The best-fit genetic disease model for rs7531806 was also an additive model ( P =5.34 × 10 −7 ). Compared with G/G , the genotype of homozygote A/A (OR Hom =1.40) showed larger OR than the heterozygote G/A (OR Het =1.10) ( Table 3 ). Table 3 Distribution of genotypes and genetic model analysis for three significant SNPs in combined samples. Full size table Gender stratification analysis These three identified SNPs were selected for stratification analysis by gender to explore the gender-related difference comparing the controls and cases, especially in the cases. However, no nominal heterogeneity was observed among the odds ratios between the male and female after stratification by gender ( Table 4 ). Table 4 Association of three SNPs with severe acne analysed by gender stratification in Chinese Han population. Full size table Both SNPs rs747650 and rs1060573 at 11p11.2 highly correlated with one another ( r 2 =1) ( Fig. 4a ). Further analysis using the 1000 genomes data set ( http://www.1000genomes.org/ ) identified another SNP, rs4237547, within the promoter region of DDB2 (damage-specific DNA binding protein 2) that also highly correlate with rs747650 ( r 2 =0.97). The Encyclopedia of DNA Elements (ENCODE, http://genome.ucsc.edu/encode/ ) data indicated that rs4237547 is located within the DNase I hypersensitivity site and transcription factor binding sites, suggesting a potential effect on gene transcription and regulation. DDB2 encodes a DNA-binding protein that is the smaller subunit of a heterodimeric protein complex and participates in nucleotide excision repair. DDB2 is critical in deciding cell fate (apoptosis or arrest) upon DNA damage [18] and mediates the ubiquitination of the histones H3 and H4 (ref. 19 ), of which H4 has been shown to be a major component in the antimicrobial action of human sebocytes [20] . DDB2 has also been identified as a novel androgen receptor-interacting protein, mediating contact with AR and the CUL4A–DDB1 complex for AR ubiquitination/degradation [21] . Consequently, speculating that DDB2 is a biological candidate gene for severe acne is not unreasonable, particularly given its involvement in androgen metabolism and inflammation processes. The SNP rs7531806 is located at the loci 1q24.2, covering a gene cluster including SELL (selectin L), SELP (selectin P) and SELE (selectin E) ( Fig. 4b ). These selectins of adhesion molecules have important roles in regulating homoeostasis and cutaneous inflammation. L-selectin is expressed on the surface of most circulating leukocytes, facilitating leukocyte migration into secondary lymphoid organs and inflammation sites. P- and E-selectin, expressed on inflamed endothelium [22] , are likewise responsible for the accumulation of blood leukocytes at sites of inflammation by mediating the adhesion of cells to the vascular lining [23] . Analysis of the gene expression profiles revealed that the mRNA expression of SELL was upregulated in acne lesions [24] . L-selectin has been shown to have an important role in mediating cutaneous inflammation by studies using gene-targeted mice [25] , [26] , [27] . Another study also reported a highly significant negative correlation between soluble L-selectin and the inflammatory disorder diffuse systemic sclerosis (dSSc) [28] . Similarly, in mice lacking both L-selectin and intercellular adhesion molecular-1 (ICAM-1) expression, the healing of wounds is delayed, probably due to the decreased leukocyte accumulation into the wound site [29] . Similarly, the absence of both P- and E-selectins markedly reduced recruitment of inflammatory cells and impaired closure of the wounds [30] . Taken together, these findings implicate a potential pathogenic role of selectins in inflammation and the scar-forming processes associated with severe acne. In summary, we carried out the first GWAS of severe acne among a Chinese population, the findings of which identified new genetic factors that may potentially contribute to severe acne susceptibility. Obviously, further fine-mapping and functional studies are warranted to determine the causal genes within the 1q24.2 and 11p11.2 loci, but the information provided herein should further our basic understanding of the pathogenesis of severe acne, serving as a jumping off point for more sophisticated and focused research efforts. Study populations We performed a two-stage GWAS. The discovery stage included 1,056 severe acne cases and 1,056 controls. The replication stage included 1,860 severe acne cases and 3,660 controls. All samples from both the discovery and replication stages were unrelated individuals of Chinese Han descent, obtained from doctors through collaboration with multiple hospitals within China. To ensure that patient and control inclusion/exclusion were done in a comparable ways across the different centres, we performed three stages of sample gathering, as follows: in the preparation stage, we created unified epidemiological surveys, which included precise criteria for the definition of a case or a control, and the standard procedures for sample collection, which included information collection, photograph taking and blood collection. Then, in the standard training stage, dermatologists from different centres were required to attend meetings for standard operation training before participant recruitment. Finally, in the sample verification stage, each sample was verified via questionnaires and photographs taken by dermatologist from First Affiliated Hospital of Kunming Medical University before its genomic DNA was extracted. The disease status of each patient and control was also reconfirmed by phone survey. All the cases of severe acne were diagnosed with grade IV according to the Pillsbury grading system, meaning that patients had many comedones and deep lesions tending to coalesce and canalize, and involving the face and the upper aspects of the trunk [6] , without systemic disorders, autoimmune diseases or chronic inflammatory diseases. Clinical information was collected from affected individuals through a full clinical checkup conducted by medical specialists. Additional demographic information was collected from cases and controls through a structured questionnaire. All controls were clinically assessed to be without acne, systemic disorders, autoimmune diseases or family history of severe acne (including first, second and third degree relatives). Given the speculated differences in genetic background between northern and southern Chinese populations [31] , the vast majority of the controls and cases for GWAS and replication studies were collected from southern Chinese populations to avoid potential population stratification. Written informed consent was obtained from each subject before sample collections, and this study was approved by the ethical committee of all participating institutions and was done in conformity with the Declaration of Helsinki and subsequent amendments. Quality control in the discovery stage The discovery stage was conducted using the Illumina HumanOmniZhongHua-8 BeadChip at the Key Laboratory of Dermatology at Anhui Medical University (Ministry of Education), Hefei, Anhui, China. We performed systematic quality control on the raw genotyping data to filter out both unqualified samples and SNPs. To evaluate the quality of the genotype data for the validation analysis, 100 randomly selected samples from the GWAS stage were re-genotyped using the Sequenom system. The concordance rate between the genotypes from the Illumina HumanOmniZhongHua-8 BeadChip and the Sequenom MassARRAY assay analyses was >99%. Samples with overall call rates of <98% were excluded from further analysis. Unexpected duplicates or probable relatives were excluded based on pairwise identity by state comparisons using the ‘PI_HAT’ value in PLINK (all PI_HAT>0.25). After filtering, 1,031 cases and 1,031 controls were retained for analysis. SNPs were excluded based on three criteria: SNPs with a call rate <98%, with minor allele frequency (MAF) <0.01 in all samples or SNPs with genotype distributions that deviated from those expected by the Hardy–Weinberg equilibrium ( P <1 × 10 −4 ) in the controls. After quality control filtering, 809,305 SNPs remained in the discovery stage. SNP selection and genotyping in replication stage SNPs for the replication stage were selected using the following criteria: SNPs with P <1 × 10 −4 for discovery samples or with P <1 × 10 −4 for gender as covariate, which might help reduce the gender effect on the results. A total of 86 SNPs that matched these criteria were accordingly included in the replication stage. We also selected 15 SNPs with nominal association evidence ( P <1 × 10 −2 in the discovery stage) that were located within or close to the nine susceptibility genes ( CD14, LIPC, MMP1, SELL, SGK1, TNC, FGFR2, WNT4 and PSTPIP1 ) with gene expression profiling evidence for acne [24] or for three syndromes with acne symptoms (Apert syndrome [32] , polycystic ovary syndrome [33] and pyogenic arthritis, pyoderma gangrenosum and acne syndrome [34] ). In total, 101 SNPs were selected for the replication. Genotyping analyses of replication were conducted by the Sequenom MassARRAY system at the Key Laboratory of Dermatology at Anhui Medical University (Ministry of Education), Hefei, Anhui, China. Quality control in replication stage We excluded SNPs with a call rate <90% or a deviation from HWE ( P <0.05) in the controls. After quality control, 87 of the previous 101 SNPs were left for further analysis. Association analysis in discovery stage In the discovery stage, we examined potential genetic relatedness based on pairwise identity by state for all of the successfully genotyped samples using PLINK 1.07 software [35] . We used PLINK 1.07 for general statistical analysis. We used the quantile–quantile plots to evaluate the overall significance of the genome-wide association results and the potential effect of population stratification. We further calculated the genomic control inflation factor and found it to be minimal ( λ GC =1.01), suggesting minimal inflation of the genome-wide association results from population stratification. The remaining samples (1,031 cases and 1,031 controls) were subsequently assessed for population outlier and stratification using a principal component analysis (PCA)-based approach. No population outliers were detected. In GWAS stage, single-marker association analyses were performed using logistic regression with gender as a covariate. The Manhattan plot of −log 10 P was generated using Haploview v4.2. Association analysis in replication and combined stage For the replication studies, 87 SNPs that passed quality control were analysed using logistic regression with gender as a covariate. Joint analysis of all combined samples of Chinese Han was conducted either by random effects model ( I 2 >25%) or by using fixed-effect model ( I 2 <25%). In addition to the allelic test of association, the genetic models (dominant, recessive and additive models) were calculated for the associated SNPs. The chi-square (χ 2 )-based Cochran’s Q statistic was also calculated to test for heterogeneity between groups in stratified analysis. The regional association plot was created using LocusZoom [36] . In stratification analysis by gender, the logistic regression analysis restricted to cases (case-only analyses) was performed with gender as the outcome variable [37] . How to cite this article: He, L. et al. Two new susceptibility loci 1q24.2 and 11p11.2 confer risk to severe acne. Nat. Commun. 5:2870 doi: 10.1038/ncomms3870 (2014).